Measurement of the intrinsic strength of crystalline and polycrystalline graphene The mechanical properties of materials depend strongly on crystal structure and defect configuration. Here we measure the strength of suspended single-crystal and bicrystal graphene membranes prepared by chemical vapour deposition. Membranes of interest are first characterized by transmission electron microscopy and subsequently tested using atomic force microscopy. Single-crystal membranes prepared by chemical vapour deposition show strengths comparable to previous results of single-crystal membranes prepared by mechanical exfoliation. Grain boundaries with large mismatch angles in polycrystalline specimens have higher strengths than their low angle counterparts. Remarkably, these large angle grain boundaries show strength comparable to that of single-crystal graphene. To investigate this enhanced strength, we employ aberration-corrected high-resolution transmission electron microscopy to explicitly map the atomic-scale strain fields in suspended graphene. The high strength is attributed to the presence of low atomic-scale strain in the carbon–carbon bonds at the boundary. Graphene exhibits exceptional mechanical [1] , [2] , [3] and electronic properties [4] , [5] , [6] which arise from its unique two-dimensional (2D) atomic structure. Chemical vapour deposition (CVD) of graphene on various metal substrates [7] , [8] , [9] provides a convenient method of scaled growth, but samples thus produced are often polycrystalline, with possible compromises to mechanical strength due to the formation of carbon structures [10] , [11] , [12] , [13] , [14] , [15] that depart from the standard honeycomb lattice of graphene. Of particular interest are the grain boundaries that form between neighbouring crystal domains in polycrystalline graphene [16] , [17] . These boundaries have been predicted to have unusual electronic [18] , thermal [19] , [20] and mechanical properties [21] , [22] , [23] that depend on the crystal orientation of individual grains as well as the exact atomic configuration at the boundary. Although recent progress on CVD graphene growth shows promise for large-scale single-crystal graphene growth [24] , [25] , [26] , [27] , [28] , it is of fundamental and practical importance to understand the effect of these structures on the properties of graphene. Recent theoretical calculations suggest that for some grain boundary configurations, a measurable transport gap may exist, allowing graphene to be used as an active component in digital electronics [18] . Interestingly, density functional theory calculations and molecular dynamics simulations predict that graphene grain boundaries can retain mechanical strengths that are comparable to single-crystal graphene [21] , [22] . Limited experimental work has been directed towards the effect of grain boundaries on electrical [29] , [30] , [31] , [32] , [33] and mechanical properties [34] , [35] of polycrystalline graphene. Although the strength of CVD graphene has been studied [16] , [34] , [35] , isolated single-crystal regions of CVD-grown graphene membranes have not been directly measured and the relationship between grain boundary orientation and failure strength of bicrystal membranes remains unknown. In addition, the critically important local atomic-scale strain field of graphene grain boundaries has not yet been measured. In this work, we measure the intrinsic strength of CVD-derived single-crystal and polycrystalline graphene. Each sample is first characterized structurally via low-voltage transmission electron microscopy (TEM) and then measured mechanically by atomic force microscopy (AFM)-induced fracture, providing a strength map of the material. We perform fracture measurements on graphene membranes comprised of single-crystal regions and bicrystal regions containing isolated grain boundaries. A nonlinear anisotropic elastic material model of graphene is implemented in finite-element analysis (FEA) simulations to understand the fracture strength of measured membranes [36] . Single-crystal membranes of CVD-grown graphene show maximum strength values comparable to previously reported values of single-crystal graphene membranes prepared by mechanical exfoliation from bulk graphite [1] . We find that graphene grain boundaries with large mismatch angles have the highest yield strengths, withstanding normal forces that approach values of single-crystal graphene. Using aberration-corrected high-resolution TEM (AC-HRTEM), we map atomic-scale strain fields at graphene grain boundaries and thereby gain insights into their remarkable strength. The strain fields are shown to be localized at the grain boundary with low strain values that are consistent with theoretical predictions. Structure mapping and mechanical testing For our studies, graphene is grown by CVD on copper foils [7] , initially characterized and subsequently transferred to a TEM support chip ( Supplementary Fig. S1 and Supplementary Methods ). Each support chip is composed of a 200 nm thick silicon nitride (SiN) window with a 50 by 50 grid of 1 μm holes on a 12 μm spacing. Once transferred and suspended, graphene membranes of interest are characterized by TEM through a combination of imaging and selected area electron diffraction (SAED) at an operating voltage of 60 kV. All membranes are initially checked to ensure that there are no unusual adsorbates, tears, holes [37] , [38] or folds [39] , [40] , which could compromise the fidelity of the measurements. Single-crystal membranes ( Fig. 1a ) contain only one crystalline region suspended over the entire 1 μm hole. Bicrystal membranes are chosen such that the graphene grain boundary separating the two different crystallographic regions is within 200 nm of the centre of the membrane. The atomic structure of a graphene grain boundary is presented in Fig. 1b with the bonds enhanced in Fig. 1c with a minimum filter [41] . When a bicrystal is identified, dark-field-TEM (DF-TEM) imaging is employed to obtain the real-space distribution of the two different crystals and the orientation of the grain boundary relative to each single-crystal region [16] , [17] . 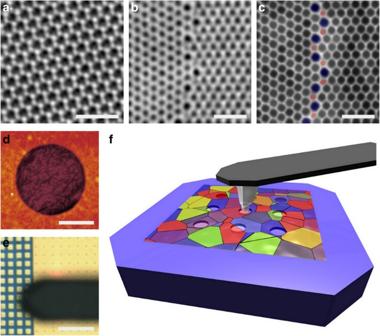Figure 1: Measuring graphene grain strength. (a) AC-HRTEM image of a single-crystal region of graphene. (b) AC-HRTEM image of a 30° graphene grain boundary stitched together with pentagon and heptagon rings (5–7 rings). (c) Image frombwith a minimal filter applied for enhanced visualization of the bond structure. The pentagons are highlighted in red and the heptagons in blue. The scale bars ina–care 0.8 nm. (d) AFM image of a suspended graphene membrane. Scale bar, 500 nm. (e) Optical microscope image of the backside of the diamond AFM probe positioned over a membrane before a fracture measurement. Scale bar, 50 μm. (f) Schematic illustration of the AFM measurement with the large-radius single-crystal diamond probe. Multicoloured tiles represent polycrystalline graphene of different orientations, which cover the perforated TEM window. Figure 1: Measuring graphene grain strength. ( a ) AC-HRTEM image of a single-crystal region of graphene. ( b ) AC-HRTEM image of a 30° graphene grain boundary stitched together with pentagon and heptagon rings (5–7 rings). ( c ) Image from b with a minimal filter applied for enhanced visualization of the bond structure. The pentagons are highlighted in red and the heptagons in blue. The scale bars in a – c are 0.8 nm. ( d ) AFM image of a suspended graphene membrane. Scale bar, 500 nm. ( e ) Optical microscope image of the backside of the diamond AFM probe positioned over a membrane before a fracture measurement. Scale bar, 50 μm. ( f ) Schematic illustration of the AFM measurement with the large-radius single-crystal diamond probe. Multicoloured tiles represent polycrystalline graphene of different orientations, which cover the perforated TEM window. Full size image Once suitable graphene membranes are identified in the TEM, the sample support chip is transferred to an AFM for imaging and mechanical testing. Membranes are first imaged using a standard high-resolution silicon tip to double check for the absence of holes or folds in the graphene membrane ( Fig. 1d ). The silicon tip is then replaced with a custom-fabricated single-crystal diamond probe with a large tip radius of 115 nm for mechanical measurements ( Supplementary Methods ). The diamond tip is required as the measured graphene membranes exhibit extremely high strength, which can damage conventional silicon AFM tips. In addition, the custom large tip is fabricated and used to ensure a uniform stress distribution over the entire region of interest. The diamond tip is positioned over a graphene membrane of interest ( Fig. 1e ) and mechanical testing is performed with a constant displacement rate towards the surface. An initial cycle of loading and unloading is performed to ensure an absence of hysteresis and graphene slippage at the membrane border. The films are then indented with the same displacement rate until a membrane fracture event occurs. A schematic illustration of the mechanical testing of polycrystalline graphene membranes suspended over holes in the TEM window with the single-crystal diamond tip is provided in Fig. 1f . TEM characterization of graphene membranes A typical bright-field TEM image and SAED pattern of a single-crystal graphene membrane is shown in Fig. 2a,b , respectively. The membranes appear as bright discs and show continuous coverage over the holes in the SiN window with no visible defects or cracks in the graphene. The diffraction pattern allows for the precise determination of the real-space orientation of the graphene crystal lattice directions. The three zig-zag (ZZ) directions of the graphene membrane shown in Fig. 2a are labelled with blue arrows on the diffraction pattern shown in Fig. 2b . Similarly, the three armchair (AC) directions of the membrane are labelled with red arrows. In this manner, it is possible to provide a compass of the crystal orientations in the graphene membranes. 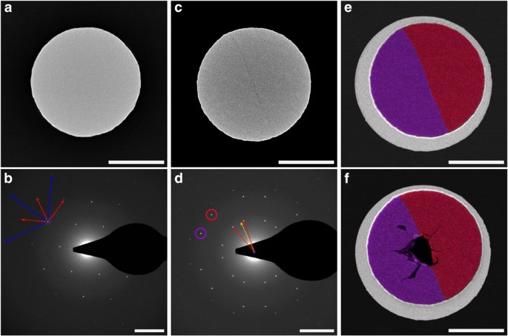Figure 2: TEM characterization of graphene membranes. (a) Bright-field TEM image of a single-crystal graphene membrane. (b) SAED pattern taken from the membrane ina. The red arrows indicate the AC lattice direction and the blue arrows indicate the ZZ lattice directions. (c) Bright-field TEM image of a bicrystal membrane. (d) SAED pattern taken from the membrane inc. The red arrows indicate the AC directions of the two different crystals. The yellow arrow shows the direction of the grain boundary. (e) Composite false colour DF-TEM image of the membrane shown incusing the two distinct diffractions spots highlighted ind. (f) Composite false colour DF-TEM image of the same membrane after fracture measurement. Scale bars ina,c,eandfare 500 nm. The scale bars inbanddare 5 nm−1. Figure 2: TEM characterization of graphene membranes. ( a ) Bright-field TEM image of a single-crystal graphene membrane. ( b ) SAED pattern taken from the membrane in a . The red arrows indicate the AC lattice direction and the blue arrows indicate the ZZ lattice directions. ( c ) Bright-field TEM image of a bicrystal membrane. ( d ) SAED pattern taken from the membrane in c . The red arrows indicate the AC directions of the two different crystals. The yellow arrow shows the direction of the grain boundary. ( e ) Composite false colour DF-TEM image of the membrane shown in c using the two distinct diffractions spots highlighted in d . ( f ) Composite false colour DF-TEM image of the same membrane after fracture measurement. Scale bars in a , c , e and f are 500 nm. The scale bars in b and d are 5 nm −1 . Full size image A complete TEM data set of a bicrystal membrane is provided in Fig. 2c–f ( Supplementary Fig. S2 ). A typical bright-field TEM image of a bicrystal is shown in Fig. 2c . The membrane appears as a bright circle in the SiN window with a dark line following the path of the grain boundary. The contrast along the grain boundary is attributed to an enhanced accumulation of adsorbates, which has been verified with AC-HRTEM imaging of similar samples prepared with identical methods. When a SAED pattern is acquired over the bicrystal membrane ( Fig. 2d ), a pattern with two distinct sets of rotated spots appears in the back focal plane of the objective lens. Figure 2e shows a false-coloured composite image of a pair of DF-TEM images formed from the collection of electrons from the two diffracted spots highlighted in Fig. 2d . The diffraction patterns reveal monolayer stitching of the two graphene grain boundaries ( Supplementary Figs S3 and S4 ). In addition, these images reveal the real-space distribution and orientation of the two different crystal regions relative to the orientation of the grain boundary. After each fracture measurement, the graphene membranes are again visualized with the TEM to understand crack propagation during failure. Figure 2f shows a false-coloured composite image of the membrane after fracture. Importantly, the crack and hole formation does not show a clear indication for propagation along the grain boundary. This likely is a consequence of graphene grain boundaries having significant line curvature at the atomic scale [16] , [17] ( Fig. 1b,c ). During a fracture measurement, a bond breakage is expected to initiate at the line defect and propagate towards the nearest defect site [22] . When a grain boundary line changes direction, however, an induced crack is expected to continue along the tangent line of the crack initiation and into the surrounding crystal grain along one of the crystallographic axis. Similar results have been observed for tears that initiate off a graphene grain boundary axis and propagate straight through the grain, with little or no propagation along the boundary [42] . The combination of SAED and DF-TEM allows for visualization of the grain boundary orientation and the independent orientations of the two crystallographic axes of the bicrystal membranes. Using this information, it is possible to understand the dependence of fracture strength on mismatch angle in the material. Here, we consider three different classes of grain boundaries: AC, ZZ and AC–ZZ. In the case of AC bicrystal membranes, the grain boundary direction lies within the angle formed between the two AC directions of each individual lattice. Figure 2c–f highlight an AC grain boundary bicrystal with the corresponding diffraction analysis. The two red arrows show the two distinct AC directions and the yellow arrow indicates the orientation of the grain boundary. The angle attributed to the grain boundary is then defined by the angle between the two AC directions. A similar analysis leads to the ZZ bicrystal classification. For the AC–ZZ membranes, the grain boundary orientation lies between one of the AC lattice directions from one grain and the ZZ lattice direction of the other grain ( Supplementary Fig. S5 ). Fracture strength measurements of graphene membranes The results of fracture force measurements on 15 single-crystal membranes and a total of 27 unique bicrystal membranes using the large radius diamond tip indenter is summarized in Fig. 3 ( Supplementary Fig. S6 ). Three exemplary force versus membrane deflection curves are shown in Fig. 3a , with the point of fracture labelled with an orange cross ( Supplementary Fig. S7 ). As expected, the single-crystal membranes (black curve) fracture at higher loading forces, whereas the bicrystal membranes have varied fracture strength which depend on the class and mismatch angle. 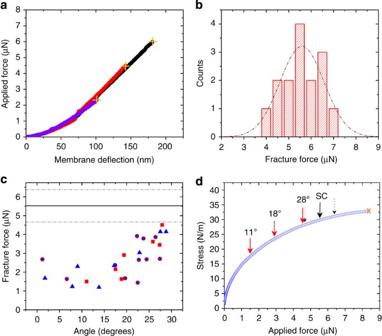Figure 3: Fracture measurements on graphene membranes. (a) Representative force versus deflection profiles for three different membranes. A single-crystal membrane is shown in black, whereas the red and purple curves belong to a large-angle AC bicrystal and a weaker AC–ZZ bicrystal, respectively. The orange cross-hairs indicate the point of fracture. (b) Histogram and Gaussian distribution of measured single-crystal fracture strength. (c) Summary of fracture force measurements on bicrystal membranes. Red squares, blue triangles and purple circles correspond to AC, ZZ and AC–ZZ bicrystals, respectively. Black and dotted lines indicate the average single-crystal fracture strength and the standard deviation about the mean, respectively. (d) 2D stress versus applied force for a theoretical single-crystal graphene membrane calculated from FEA simulations. Black arrow indicates the average measured single-crystal fracture force and dotted arrows show the standard deviation. Red arrows highlight the trend of decreased strength with decreasing mismatch angle for AC grain boundary bicrystals. Figure 3: Fracture measurements on graphene membranes. ( a ) Representative force versus deflection profiles for three different membranes. A single-crystal membrane is shown in black, whereas the red and purple curves belong to a large-angle AC bicrystal and a weaker AC–ZZ bicrystal, respectively. The orange cross-hairs indicate the point of fracture. ( b ) Histogram and Gaussian distribution of measured single-crystal fracture strength. ( c ) Summary of fracture force measurements on bicrystal membranes. Red squares, blue triangles and purple circles correspond to AC, ZZ and AC–ZZ bicrystals, respectively. Black and dotted lines indicate the average single-crystal fracture strength and the standard deviation about the mean, respectively. ( d ) 2D stress versus applied force for a theoretical single-crystal graphene membrane calculated from FEA simulations. Black arrow indicates the average measured single-crystal fracture force and dotted arrows show the standard deviation. Red arrows highlight the trend of decreased strength with decreasing mismatch angle for AC grain boundary bicrystals. Full size image Force measurements on single-crystal membranes reveal that single-crystal graphene synthesized by CVD has strength which is comparable to single-crystal graphene isolated by mechanical exfoliation [1] . The distribution of fracture forces for 15 single-crystal membranes is shown in Fig. 3b . The average measured fracture force is 5.52 μN with a standard deviation of 0.86 μN. From FEA simulations of the indentation process we calculate the stresses and strains at failure for a given fracture force ( Supplementary Fig. S8 ). For a measured force of 5.52 μN we calculate the maximum 2D stress at failure to be 30 N m −1 . For graphene with a thickness of 0.335 nm, the 3D stress at failure is 90 GPa. The strongest single-crystal membrane fails at a fracture force of 6.8 μN with a derived 2D stress of 31.5 N m −1 , which yields a 3D stress of 94 GPa. The stresses at failure of 90 and 94 GPa are close to our theoretically calculated maximum stress at failure of 98 GPa for strain along the ZZ and AC directions of simulated single-crystal graphene membranes. Fracture force measurements on bicrystal graphene membranes reveal that large-angle ZZ and AC grain boundaries have strength approaching that of single-crystal graphene. The large-angle grain boundary membranes show fracture forces that are as high as 4.5 μN with many membranes failing at forces around 4.0 μN. From our FEA simulations we find that the maximum 3D stress at failure is ~83 GPa for the strongest large angle grain boundary and 80 GPa for the others. Remarkably, these large-angle grain boundaries have strengths that are 89–92% of the strength of single-crystal graphene membranes. As the mismatch of the two different bicrystal lattices decreases, a decrease in fracture strength is observed. For the lowest angle mismatches, we observe fracture forces around 1.5 μN. These fracture forces correspond to a maximum stress at failure of 53 GPa, which is 59% of the average single-crystal membrane stress at failure. The AC—ZZ membranes show varied strength, with the highest fracture forces between 71 and 69% of the average single-crystal membrane value. These membranes have derived 3D strengths of approximately 77 GPa. Atomic-scale strain mapping of graphene grain boundaries To understand the enhanced strength of graphene grain boundaries, we use AC-HRTEM to determine the precise atomic configuration at a local region of a grain boundary and map the local strain fields present in each lattice of the bicrystals, for nominally externally unstressed membranes. 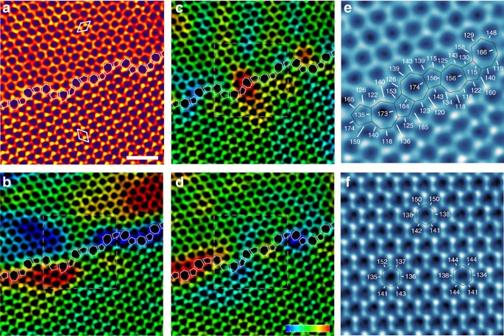Figure 4: Strain at graphene grain boundaries. (a) TEM image of a 30° graphene grain boundary. White diamonds show the unit cells of the two different crystal lattices with the white heptagons and pentagons highlighting the grain boundary stitching. The scale bar is 0.8 nm. (b–d) The perpendicular (εyy), parallel (εxx) and shear (εxy) strain field maps of the grain boundary ina, respectively. (e) Bond lengths of the grain boundary region enclosed by the dashed box inb–d. (f) Bond lengths of a single-crystal region of graphene. The colour scale forb–dis shown ind, with a range of −5% (blue) to +5% (red) strain with white tick labels every 1% strain. Figure 4a shows an AC-HRTEM image of a local region of a large-angle, 30 degree, grain boundary. The most prominent feature is the complete stitching of the two lattices with alternating pentagon and heptagon rings (5–7 rings). Recent theoretical calculations suggest that the exact atomic arrangement and corresponding strains surrounding collections of 5–7 rings ultimately determine the yield strength of graphene grain boundaries [21] , [22] . By comparing the atomic positions at the boundary with the expected positions derived from the surrounding lattices of each crystal, we map the perpendicular ( ε yy ), parallel ( ε xx ) and shear (ε xy )strain fields ( Fig. 4b–d , respectively). In each of the strain field maps there exist regions at the grain boundary that exhibit negligible strain. In particular, the central region of the grain boundary image reveals that the two lattices stitch well together with strains comparable to the surrounding single-crystal regions. Figure 4: Strain at graphene grain boundaries. ( a ) TEM image of a 30° graphene grain boundary. White diamonds show the unit cells of the two different crystal lattices with the white heptagons and pentagons highlighting the grain boundary stitching. The scale bar is 0.8 nm. ( b – d ) The perpendicular ( ε yy ), parallel ( ε xx ) and shear ( ε xy ) strain field maps of the grain boundary in a , respectively. ( e ) Bond lengths of the grain boundary region enclosed by the dashed box in b – d . ( f ) Bond lengths of a single-crystal region of graphene. The colour scale for b – d is shown in d , with a range of −5% (blue) to +5% (red) strain with white tick labels every 1% strain. Full size image The stitching of the two lattices is accomplished via pentagon-heptagon (5–7) rings with bond lengths near the ideal bond lengths of graphene ( Fig. 4e ). In single-crystal regions of the graphene membranes ( Fig. 4f ), the bond lengths vary between 134 and 152 pm with an average of 142 pm and a standard deviation of 5pm. This matches well with the expected value of 143 pm and is consistent with previous reports of measured bond length variations of single-crystal regions of monolayer graphene imaged under similar conditions [13] . The uncertainty in measured bond lengths may be the result of a combination of possible contributing factors, which include lateral drift in the sample stage, a combination of tilting and mechanical vibration, or local phonon excitations to the lattice by the illuminating beam [43] . In the central region of the grain boundary, the bond lengths vary between 115 and 185 pm, with many of the individual bonds having lengths within the range of the single-crystal regions of graphene. The maximum compressive (blue) and tensile (red) strain present at the boundary is approximately 6%, with the strain being most prominent in the ε yy strain field. The strain fields are localized at the 5–7 rings of the grain boundary and dissipate at a maximum distance of approximately 1.75 nm. In single-crystal regions of graphene, the average measured strain is 0% with a deviation of 0.209–0.326%, which provides confidence in the measured strain at the grain boundary ( Supplementary Figs S9–S12 ). Although the presented strain analysis does not include possible local warping or rippling [41] , [44] , [45] of the graphene lattices, the tensile strain due to apparent bond elongation cannot be due to local tilting of the graphene lattice and is attributed to real strain in the lattice [13] . In recent density functional theory calculations and molecular dynamics simulations it is shown that strains of 5.4% are expected to be present in large-angle grain boundaries and still maintain strengths comparable to a single-crystal graphene sheet [21] . As graphene sheets can tolerate local strains near the 6% strain we observe, we expect that the large-angle bicrystals present in the fracture force experiments exhibit similar local strains at the grain boundary of the individual crystals. In summary, we have measured the fracture strength of suspended single-crystal and bicrystal graphene membranes of polycrystalline graphene. Using SAED and low-voltage TEM imaging, we are able to identify membranes of interest and perform strength measurements using a custom-fabricated large radius diamond probe in an AFM. Using a nonlinear anisotropic elastic model of graphene [36] , in combination with FEA simulations, we determine that single-crystal graphene membranes grown by CVD have strengths comparable to graphene prepared by mechanical exfoliation from bulk graphite [1] . Bicrystal membranes with large-angle grain boundaries show enhanced strength when compared with similar low-angle grain boundaries. Large-angle grain boundaries fail at stresses that are as high as 92% of their single-crystal counterparts. In addition, we map the atomic-scale strain fields present at graphene grain boundaries using AC-HRTEM. The enhanced strength of large-angle grain boundaries is attributed to the low strains observed in the carbon–carbon bonds of the boundary. This work suggests that carbon structures that depart from the standard hexagonal bonding of graphene may be used to produce a new class of ultra-strong 2D materials. In addition, the experimental techniques outlined in this work can easily be used to study the strength of other 2D polycrystalline materials, such as CVD hexagonal boron nitride (h-BN) and molybdenum disulphide (MoS 2 ), to further our understanding of this new class of materials. Structural characterization in a TEM All TEM work done on samples for mechanical strength measurements is accomplished at a low operating voltage of 60 kV in an FEI Technai T12 TEM. DF-TEM images are acquired with exposures between 10 and 20 s. Each diffraction spot of two distinct graphene grains of each bicrystal is imaged with the dark-field mode to ensure that the membranes were comprised of two distinct regions. The SAED patterns are checked to ensure that each bicrystal graphene membrane was comprised of two fused monolayer regions. Fracture force determination in an AFM Fracture measurements are performed in a Bruker AXS Dimension Icon AFM with a closed loop scan head. The spring constant calibration of the cantilever is accomplished by approaching the diamond tip onto a reference cantilever with a known spring constant and performing a series of force spectroscopy measurements. After calibration, the tip is used to image the membrane of interest to find the position of indentation. The tip is allowed to load and unload the surface with small displacements to ensure no hysteresis in the measurement. Last, the tip is allowed to press into the membranes at a loading rate of 1 Hz over a piezo sweep distance of 600 nm. The subsequent graphene membrane deflection is obtained by subtracting the tip deflection measured at the photo diode from the z -piezo displacement. FEA of graphene fracture strength The indentation of graphene is simulated with a finite-element implementation of nonlinear membrane elasticity based on finite-deformation (large-strain) kinematics. The stress–strain response of graphene is modelled by a fifth-order anisotropic strain energy [36] . Meshes of 10,981 nodes and 5,400 quadratic triangular elements with C 0 -Lagrange interpolation are used for the simulated membrane. Contact between the membrane and a rigid indenter was modelled as frictionless, and enforced with a standard Augmented-Lagrange constraint implementation. Fixed displacement boundary conditions are imposed along the circular boundary, and indentation forces are applied via displacement control. The nonlinear finite-element equilibrium equations are solved by the iterative Quasi-Newton L-BFGS-B method. The membrane failure (ultimate force at fracture) is estimated by the state in which the nonlinear solver diverged. AC-HRTEM of grapheme All AC-HRTEM images of graphene were acquired using TEAM 0.5 at the National Center for Electron Microscopy (NCEM) in Lawrence Berkeley National Laboratory (LBNL). The microscope is a modified FEI Titan microscope with a high brightness Schottky-field emission gun, monochromator and spherical aberration corrector. The microscope is operated at 80 kV with the monochromator turned on to provide an energy spread of ~0.11 eV. Images were acquired with exposures of 4 s, which provided high signal-to-noise and minimal image blur due to sample drift. Real-space strain measurements in graphene grain boundaries We determine the initial atomic positions from intensity peaks in the micrograph. The peak positions are refined by fitting 2D Gaussian functions to each position simultaneously. Best-fit lattices for each grain are computed using linear regression. At the grain boundary, each atomic position is assigned to the grain that had the closest ideal lattice position. For each atomic position, displacement vectors are defined as the deviation from the ideal lattice positions. These measurements are resampled into continuous 2D displacement maps using Gaussian kernel density estimation with a bandwidth equal to the unit cell length. Last, the perpendicular ( ε yy ), parallel ( ε xx ) and shear ( ε xy ) strain maps are calculated by numerical differentiation of the displacement maps. The parallel direction ( x -direction) of the grain boundary in Fig. 4 was set to the crystallographic orientation closest to the grain boundary. The grain boundary is tilted ~3° from the x -direction, and the grain boundary has a perfect 30° misorientation within the accuracy of the AC-HRTEM measurement. How to cite this article: Rasool, H. I. et al. Measurement of the intrinsic strength of crystalline and polycrystalline graphene. Nat. Commun. 4:2811 doi: 10.1038/ncomms3811 (2013).